Giant cationic polyelectrolytes generated via electrochemical oxidation of single-walled carbon nanotubes Previously, reduced single-walled carbon nanotube anions have been used for effective processing and functionalization. Here we report individually separate and distinct (that is, discrete) single-walled carbon nanotube cations, directly generated from a pure anode using a non-aqueous electrochemical technique. Cyclic voltammetry provides evidence for the reversibility of this nanoion electrochemisty, and can be related to the complex electronic density of states of the single-walled carbon nanotubes. Fixed potentiostatic oxidation allows spontaneous dissolution of nanotube cations (‘nanotubium’); Raman spectroscopy and transmission electron microscopy show that sequential fractions are purified, separating amorphous carbon and short, defective single-walled carbon nanotubes, initially. The preparation of nanotubium, in principle, enables a new family of nucleophilic grafting reactions for single-walled carbon nanotubes, exploited here, to assemble nanotubes on amine-modified Si surfaces. Other nanoparticle polyelectrolyte cations may be anticipated. Fullerenes can be (electro)chemically reduced or oxidized to generate isolated fulleride (C 60 x− , x =1–7) and fullerenium (C 60 x+ , x =1–3) ions, respectively [1] , [2] . The analogous processes for larger nanoparticulate carbons rather than clearly molecular carbon species has attracted growing interest in recent years, but so far via reduction only. In particular, charging provides a means to process single-walled carbon nanotubes (SWCNTs), whilst avoiding aggressive sonication and time consuming centrifugation processes. Anionic nanotube (nanotubide) polyelectrolytes have been generated using reductive chemical (alkali metal naphthalide/THF [3] , alkali metal/liquid ammonia [4] , [5] ) and electrochemical approaches [6] . The covalent chemistry of reduced carbon nanomaterials has also been studied extensively, extending to a whole library of electrophilic addition and radical-based surface modifications [7] , [8] , [9] that can be tailored to specific applications. The logical corollary, namely oxidation of SWCNTs to generate SWCNT n+ is an intriguing possibility, and may serve as a model for the generation of other large nanoparticulate polyelectrolyte cations. By analogy to fullerenium, the term ‘nanotubium’ is proposed for cationic SWCNT polyelectrolytes. Chemically, only superacids, such as chlorosulfonic acid, are reported [10] to generate sufficient positive charge density for spontaneous dissolution of SWCNTs, although, in this case, via reversible proton transfer. Based on initial evidence, superacids are proposed to generate a polarized SWCNT-H + moiety rather than permanently remove electrons from the SWCNTs by hydrogen evolution, or covalent C–H bond formation. Very recently, a purely electrochemical reduction [6] was shown to generate nanotubide species (SWCNT n- ) in polar aprotic solvents containing alkali metal or tetrabutylammonium cations. At reducing potentials beyond −1.6 V versus Ag/Ag + , dissolution of discrete, individualized, nanotubide anions was observed; complete dissolution of commercial HiPco and CoMoCAT SWCNTs was achieved at a potential of −2.3 V versus Ag/Ag + . This success relied on the use of reductively stable electrolytes, low ionic concentrations to minimize electrostatic screening and ultra-dry conditions. In order to extend this strategy to the electrochemical oxidative dissolution of individualized nanotubium ions, different electrolyte systems are required that are more stable to oxidation. After considering a range of options, electrolytes based on the hexafluoroarsenate anion (AsF 6 − ) dissolved in cyclic carbonates such as propylene carbonate (PC) were selected, owing to their relatively good oxidation stability [11] . These electrolytic solutions were found to be completely stable up to ~+1.6 V versus Ag/Ag + , but not higher, making the extended study of electrochemical SWCNT oxidation more challenging than equivalent reductions. Nevertheless, this study shows that, using potentiostatic electrochemical oxidation, it is possible to dissolve individualized nanotube cations; the possibility of subsequent nucleophilic addition reactions is illustrated with a surface assembly reaction. Generation of nanotubium dispersions The cyclic voltammetry (CV) of commercial CoMoCAT65 SWCNTs performed under oxidative potentials, in 0.1 M LiAsF 6 /PC, can be overlaid ( Fig. 1 ) with the data obtained for their reduction, in 0.1 M NaClO 4 /DMF. The central region (−0.5 V to +0.5 V), showing lower total capacitance, relates to the semiconducting SWCNTs; the ~1.0 V band gap corresponding to the first reduction and oxidation events of the most abundant (6,5) species in the sample, similar to effects identified in (6,5) SWCNT chemical doping experiments [12] (see Supplementary Fig. S1 ). The different shapes of the oxidative and reductive voltammograms are due to the different intercalant ion sizes (Na + versus AsF 6 − ). The redox features are better defined for the negative potential range, upon the intercalation of smaller Na + ions. Although the size of the counter ion may have a subtle effect on the dissolution process, in accordance with polyelectrolyte theory [13] , charging appears broadly symmetric about the Fermi level. 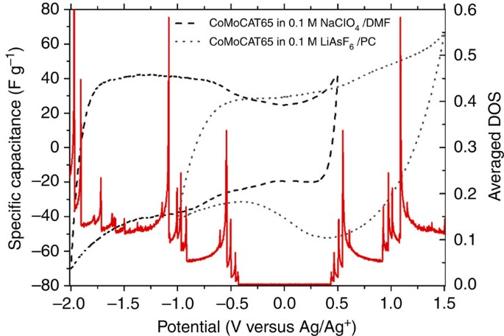Figure 1: Cyclic voltammetry of an as-received CoMoCAT65 powder electrode. The combined reduction and oxidation cycles in 0.1 M NaClO4/DMF and 0.1 M LiAsF6/PC, respectively, at a scan rate of 0.5 mV s−1. The averaged DOS for the CoMoCAT65 powder, weighted by the relative proportion of(n,m)species is overlaid in red (seeSupplementary Fig. S1for derivation). A control CV for the oxidative cycle without SWCNTs present is shown inSupplementary Fig. S2. Figure 1: Cyclic voltammetry of an as-received CoMoCAT65 powder electrode. The combined reduction and oxidation cycles in 0.1 M NaClO 4 /DMF and 0.1 M LiAsF 6 /PC, respectively, at a scan rate of 0.5 mV s −1 . The averaged DOS for the CoMoCAT65 powder, weighted by the relative proportion of (n,m) species is overlaid in red (see Supplementary Fig. S1 for derivation). A control CV for the oxidative cycle without SWCNTs present is shown in Supplementary Fig. S2 . Full size image As-synthesized nanotube powders typically contain a large proportion of amorphous carbon, metal catalyst and other graphitic debris as well as the desirable nanotubes themselves. SWCNTs do not readily dissolve in the electrolyte even with prolonged bath sonication (12 h). Holding the electrochemical potential at constant positive potentials greater than +1.4 V versus Ag/Ag + leads to the intercalation of AsF 6 − ions into the powder electrode, followed by swelling, exfoliation/debundling and diffusion of nanotubium species away from the powder bed, once charge repulsion overcomes the significant attractive van der Waals surface interactions ( Fig. 2a–c ). The initiation time (before observable dissolution) corresponds to charging of the powder to ~1 charge/100 C atoms. The charge density is equivalent to that found for electrochemical reduction, [6] as expected given the symmetric density of states (DOS) near the Fermi level. Owing to the relatively high viscosity [14] of the PC solvent (~2.5 cP at 25 °C), the nanotubium polyelectrolyte formed a concentration gradient perpendicular to the original powder bed; different fractions from this solution were analysed by transmission electron microscopy (TEM) and Raman spectroscopy. 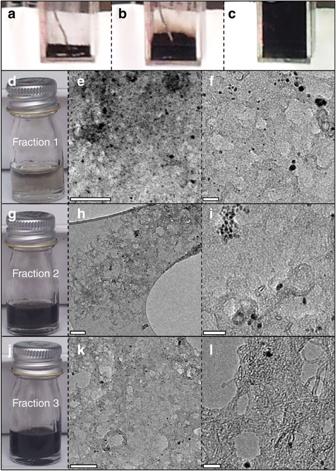Figure 2: Spontaneous electrochemical dissolution of nanotubium species. (a–c) Photographs showing the spontaneous dissolution of SWCNTn+under potentiostatic control in 1 mM LiAsF6/PC, +1.6 V versus Ag/Ag+for 120 h. Fractions were collected at different distances from the working electrode. (d) Photograph and (e,f) TEM images of fraction 1. (g) Photograph and (h,i) TEM images of fraction 2. (j) Photograph and (k,l) TEM images of fraction 3. The presence of significant amounts of metal catalyst and amorphous/defective materials is apparent in the top fraction (fraction 1). A high degree of SWCNT individualization/debundling is observed in the lower fraction (fraction 3). (e) Scale bar, 100 nm; (f) Scale bar, 20 nm; (h) Scale bar, 100 nm; (i) Scale bar, 20 nm; (k) Scale bar, 100 nm; (l) Scale bar, 10 nm. Figure 2: Spontaneous electrochemical dissolution of nanotubium species. ( a – c ) Photographs showing the spontaneous dissolution of SWCNT n+ under potentiostatic control in 1 mM LiAsF 6 /PC, +1.6 V versus Ag/Ag + for 120 h. Fractions were collected at different distances from the working electrode. ( d ) Photograph and ( e,f ) TEM images of fraction 1. ( g ) Photograph and ( h,i ) TEM images of fraction 2. ( j ) Photograph and ( k , l ) TEM images of fraction 3. The presence of significant amounts of metal catalyst and amorphous/defective materials is apparent in the top fraction (fraction 1). A high degree of SWCNT individualization/debundling is observed in the lower fraction (fraction 3). ( e ) Scale bar, 100 nm; ( f ) Scale bar, 20 nm; ( h ) Scale bar, 100 nm; ( i ) Scale bar, 20 nm; ( k ) Scale bar, 100 nm; ( l ) Scale bar, 10 nm. Full size image Characterization of the nanotubium dispersions TEM of the nanotubium dispersions ( Fig. 2 ) was challenging due to the presence of electrolytic salts that had to be removed by washing before imaging. Nevertheless, a distinct change in sample purity between the different fractions was observed; the top fraction (Fraction 1) typically contained predominantly metal catalyst particles and defective carbonaceous species. The lower fractions contained increasing concentrations of individualized nanotubes with fewer metal catalyst impurities. Assuming that the oxidative and reductive processes are symmetric, the result can be compared with the preferential dissolution of defective material observed after equilibrating at relatively modest reducing potentials [6] . Thus, although differential diffusion may have a role in the current experiments, the segregation is likely to be driven by selective charging and dissolution. A dissolution yield (~21 wt%) was estimated from UV–vis absorption measurements of the combined middle and bottom fractions; the top fraction was not included as it contained only a low concentration, predominantly of non-nanotube materials. Unfortunately, the maximum available electrode potential does not yet allow the charge densities required for complete SWCNT dissolution on the reductive side. At more positive potentials (> +1.6 V), further dissolution should be observed, but once the stability of the electrolyte is exceeded, SWCNT functionalization via electrolyte degradation cannot be excluded. Raman spectra ( Fig. 3 ) of SWCNTs show characteristic features that semi-quantitatively relate to sample purity, defect concentration, electronic type and diameter distribution. The Kataura plot and published data [15] , [16] were used to assign the helicities ( n,m ) of nanotubes present in a particular sample. Radial-breathing modes (RBMs) are not present for charged nanotubium species ( Supplementary Fig. S3 ) due to the extensive charging which bleaches the resonant absorption of the primary laser [17] ; as the charge is quenched upon exposure to air, the RBMs are gradually and fully restored to the RBMs of the dissolved fraction after ~3 h, suggesting no damage or functionalization. The G (~1,600 cm −1 ) and D peaks (~1,350 cm −1 ) are related to structural order (sp 2 carbon) and disorder (sp 3 carbon), respectively; the relative intensities of these peaks ( I D / I G ) is useful for comparing the defect concentration across different samples. The consistent increase in I D / I G ratio from fraction 3 to fraction 1, for both laser excitations ( Fig. 3a ), complements the segregation of amorphous/defective material observed in TEM ( Fig 2 ). The degree of charging required to dissolve the nanotubium ions was estimated to be ~1 charge/60 C atoms. The I D / I G ratios obtained are also comparable to those observed at the corresponding stage of the reductive dissolution for HiPco SWCNTs, which did not involve functionalization. The laser excitations used (1.96 and 2.33 eV), resonate with the optical transitions of a mixture of semiconducting and metallic nanotubes. At E laser =1.96 eV, RBM peaks originate from larger diameter metallic nanotubes (>1 nm) and smaller diameter semiconducting tubes (0.7–1 nm). Complementary RBM signals from the dissolved and undissolved fractions indicate some selectivity in the dissolution process, with apparently large diameter or metallic species dissolved preferentially, as shown previously in reductive chemical charging experiments [5] , [8] . Further confirmation by UV–vis-nIR absorption spectroscopy will require larger-scale processing and improved sample purities. 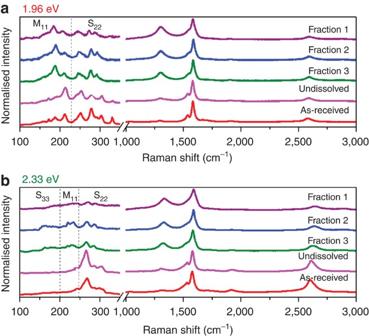Figure 3: Raman spectroscopic characterization. Raman spectra of the dissolved nanotubium fractions (1–3), the undissolved CoMoCAT65 powder and as-received CoMoCAT65 powder using excitation energy (wavelength) (a)Elaser=1.96 eV (633 nm) and (b)Elaser=2.33 eV (532 nm). RBM assignments of the Raman spectra (as-received CoMoCAT65 powder) are labelled. The RBM regions ina,bare normalized to the total RBM intensity of each fraction. The spectra were obtained by averaging five measurements on different locations of the drop-cast film. Figure 3: Raman spectroscopic characterization. Raman spectra of the dissolved nanotubium fractions (1–3), the undissolved CoMoCAT65 powder and as-received CoMoCAT65 powder using excitation energy (wavelength) ( a ) E laser =1.96 eV (633 nm) and ( b ) E laser =2.33 eV (532 nm). RBM assignments of the Raman spectra (as-received CoMoCAT65 powder) are labelled. The RBM regions in a , b are normalized to the total RBM intensity of each fraction. The spectra were obtained by averaging five measurements on different locations of the drop-cast film. Full size image Nanotubium reactivity True nanotubium ions might be expected to react via a set of pathways related to those summarized for fullerenium cations by Bohme [18] . The successful addition of ammonia, aliphatic amines, nitrogen heterocycles, protons, nitriles, water, alcohols, carbonyl compounds (carboxylic acids, ketones, aldehydes, esters), cyclic aliphatic oxides, alkenes and Diels-Alder reagents (for example, dienes, polycyclic aromatic hydrocarbons) as well as iron pentacarbonyl to fullerenium cations indicates a wide range of chemistries that may also be available to nanotubium species. In contrast, the reaction of nucleophiles with superacid-dissolved SWCNTs tends to lead to deprotonation; for example, the addition of water is reported to regenerate neutral SWCNTs without the occurrence of any permanent oxidation or other functionalization [10] . Interestingly, C 60 ·+ is sufficiently reactive that the counterions of most superacids (excepting those based on carboranes) directly attack as nucleophiles; higher fullerenes, such as C 76 , are more tractable as their cations have lower oxidation potentials [1] , [19] . The presence of nanotubiums and their reactivity towards nucleophiles was confirmed using silicon wafers functionalized with (3-aminopropyl)triethoxysilane (APTES) [20] . Dry wafers were soaked in the dissolved nanotubium fraction, under N 2 , then air-quenched and washed successively with PC, water and ethanol in order to remove the remaining soluble electrolyte/undeposited materials from the surface and confirm successful covalent addition of the amine groups to the nanotube surface ( Fig. 4 ). Control experiments exposing methyl-grafted silicon to nanotubium, and amine-grafted silicon to a neutral nanotube dispersion sonicated in NMP showed no sign of individually deposited SWCNTs, after similar washing (see Supplementary Fig. S4 ). AFM images ( Fig. 4 ) of the nanotubium-soaked APTES-treated wafers show individualized SWCNTs with diameters 0.5–1.1 nm and average length distribution 100–150 nm. Particulate impurities, dissolved during the electrochemical process (see TEM, Fig. 2 ), are also present. Interestingly, there appear to be some regions of SWCNT alignment. Until the process is scaled to macroscopic quantities in solution, it is difficult to confirm the final modified SWCNT structure and possible by-products, in detail, however, the alignment of nanotubes may be effected by two possible electrostatically driven mechanisms. (i) a reversible reaction that allows restructuring of the surface, for example, by the generation of an ammonium cation in an analogous manner to fullerenium chemistry [18] , or (ii) liquid crystalline ordering at the deposition interface due to high localized SWCNT concentrations [21] . 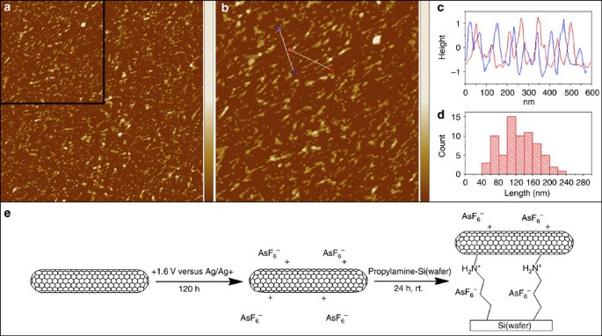Figure 4: Reactivity of nanotubium species. (a) AFM image of nanotubium species deposited on an APTES-functionalized silicon substrate (XandYscale, 5 μm;Zscale, 0–10 nm). (b) Enlarged area of the region highlighted by the black box in a (XandYscale, 2.5 μm;Zscale, 0–10 nm). (c) Height analysis of two selected cross-sections in b. (d) Length analysis of 70 SWCNTs identified fromb. (e) Proposed scheme for the reaction between nanotubium species and amines present on the silicon surface (based on ref.17). Figure 4: Reactivity of nanotubium species. ( a ) AFM image of nanotubium species deposited on an APTES-functionalized silicon substrate ( X and Y scale, 5 μm; Z scale, 0–10 nm). ( b ) Enlarged area of the region highlighted by the black box in a ( X and Y scale, 2.5 μm; Z scale, 0–10 nm). ( c ) Height analysis of two selected cross-sections in b. ( d ) Length analysis of 70 SWCNTs identified from b . ( e ) Proposed scheme for the reaction between nanotubium species and amines present on the silicon surface (based on ref. 17 ). Full size image Discrete nanotubium cations can be elegantly prepared electrochemically by direct electron transfer; the spontaneous dissolution without agitation, and the reversible CV, indicates a thermodynamic equilibrium process. The electrochemical dissolution and electrodeposition of these intriguing giant cations raises interesting fundamental questions about the nature of nanoparticle polyelectrolytes and electrochemical electron transfers that involve a large number of electrons per ion. The combination of oxidative and reductive electrochemistry provides a very wide potential window over which the electronic properties of SWCNTs can be probed. As more monodispersed materials become available, through iterated electrochemical processing, or otherwise, the underlying phenomenology will be studied in more detail. The electrochemical approach offers practical benefits for dissolving, purifying and potentially sorting individual SWCNTs, without the damaging processes of conventional purification chemistry or ultrasound; in the long run, the method may be as scalable as other electrochemical processes widely used industrially for electrowinning, including in inert atmospheres. The initial fractions dissolved contain a high proportion of short SWNTs, which may be attractive in certain applications. At the present stage, the maximum electrode potentials possible (without electrolyte degradation and subsequent unwanted functionalizations) are sufficient to observe small quantities of individualized SWCNT cations; future studies will exploit different solvent mixtures, solvent/electrolytic salt combinations or ionic liquids to extend the oxidative stability in order to scale the process for further chemical studies or potential device applications. Perhaps most interestingly, the electrochemical oxidation of SWCNTs opens up a whole new library of functionalizations based on nucleophilic additions and radical reactions, previously reported for fullerenium species. Although both require counteranions, the nature of the charge is quite distinct for nanotubium species (hole injection) compared with superacid-dissolved SWCNTs (protonation), implying different reactivity. This first success with nanotube cations suggests that a whole class of other nanoparticle cations might be prepared electrochemically, as long as the particles have sufficient integrity, electrochemical stability and electrical conductivity. The availability of these charged species offers the possibility of electrostatically-driven assembly and manipulation, including the purification of heterogeneous mixtures. In the context of nanocarbons, this challenge is a major obstacle to the successful study of fundamental properties and implementation of devices. The extent to which oxidation and reduction processes are indeed equivalent or offer characteristic advantages remains to be fully explored. Materials CoMoCAT SWCNTs (Batch: SG65-37; SWeNT, USA) were used as-received without any further purification treatments. N,N -Dimethylformamide/DMF (anhydrous, 99.8%), propylene carbonate/PC (anhydrous, 99.7%), 1,2-dichlorobenzene/DCB (anhydrous, 99%), chloroform (≥99.5%), N -methylpyrrolidone (anhydrous, 99.5%), 2-propanol/IPA (≥99.8%), sodium perchlorate (NaClO 4 ), lithium hexafluoroarsenate (LiAsF 6 ), APTES (≥98%) and triethoxymethylsilane (99%) were all purchased from Sigma-Aldrich and used as-received. Electrolytic solutions were further dried by 3 or 4 Å molecular sieves and stored in a glove box. Platinum wire electrodes (laboratory reagent, 0.5 × 100 mm 2 ) were purchased from Fisher Scientific (Loughborough, UK), platinum foil (99.95% purity, 0.125 × 25 × 25 mm 3 ) and silver wire (99.99% purity, 0.25 mm × 25 m) were purchased from Advent Research Materials (Oxford, UK). The reference electrode, Ag/Ag + , and counter electrode parts (sample holders (6 mm O.D. ), porous Vycor frits (2.85 mm O.D.) and heat-shrink PTFE tubing) were all purchased from IJ Cambria Scientific (Llanelli, UK). Electrochemical cell setup The electrochemical cell was custom designed and produced by an in-house glassblower [5] . Approximately 7 mg CoMoCAT powder was placed at the bottom of the electrochemical cell, on top of a 10-mm 2 piece of platinum foil attached to a platinum wire. The electrochemical cell was sealed and connected to a Schlenk line for drying of the SWCNTs and glassware in vacuo (250 °C, 30 min, then room temperature, overnight). The electrochemical cell was transferred to the glove box, and pre-dried electrolytic solutions added (1 mM (dissolution) or 0.1 M (CV) salt/solvent dried over 3 or 4 Å molecular sieves, 3–7 days). The reference electrode, Ag/Ag + , contained 0.01 M silver nitrate and 0.1 M TBAP in acetonitrile. A porous glass frit protected platinum wire counter electrode was used throughout to ensure no by-products entered the working electrode compartment. The counter electrode compartment contained ~1 M salt/solvent. The electrochemical cell remained sealed throughout the experiments in case of glove box contamination. After the reaction, the dissolved SWCNT fractions were removed from the electrochemical cell by syringe for subsequent characterization. Preparation of aminopropyl modified silicon wafer Silicon substrates (Agar Scientific, UK) were cleaned by dipping into a freshly prepared piranha solution (H 2 SO 4 -H 2 O 2 2:1 v/v) at 100 °C for 15 min followed by rinsing thoroughly with de-ionized water. Cleaned substrates were then dried under a stream of nitrogen. The addition of APTES to silicon wafer surface was carried out at 110 °C under nitrogen. A freshly cleaned silicon substrate was immersed in a 10 −2 M solution of APTES in anhydrous DCB (20 ml) for 16 h. The substrate was removed, sonicated 5 min in DCB (2 × 10 ml) then in chloroform (2 × 10 ml) and blown with dry nitrogen. Preparation of methyl modified silicon wafer Silicon substrates were cleaned as described above and reacted with 10 −2 M solution of triethoxymethylsilane in anhydrous DCB (20 ml) for 16 h at 110 °C. The substrate was removed, sonicated for 5 min in DCB (2 × 10 ml) then in chloroform (2 × 10 ml) and blown with dry nitrogen. AFM sample preparation SWCNT n+ functionalization. Vacuum-dried APTES-modified silicon substrates were soaked horizontally in nanotubium dispersion (~0.1 mg ml −1 from a mixture of all fractions) in a nitrogen glove box overnight. The substrate was removed from the glove box, sonicated (VWR ultrasonic cleaning bath, 80 W) in PC (5 ml, 15 s), water (5 ml, 15 s) and ethanol (5 ml, 15 s) successively, and vacuum dried at room temperature. Control sample preparation. Sample a: vacuum-dried methyl-modified silicon substrate was horizontally soaked in nanotubium dispersion in the glove box overnight before removal and washing using the above procedures. Sample b: ~15 mg as-received SWCNTs were dispersed in 15 ml NMP using ultrasonic processor (150 W, 2 h) followed by ultracentrifugation (120,000 g , 30 min). The supernatant was removed and the aminopropyl modified silicon wafer soaked horizontally in this dispersion overnight before removal and washing using the above procedures. Equipment A Solartron SI1287 Potentiostat (Solartron Analytical, UK) was used for electrochemical measurements using CorrWare 2 software. All experiments were conducted in an mBraun Labmaster SP glove box. Levels of moisture and oxygen were <1 p.p.m. throughout the duration of all electrochemical experiments. Estimates of charge/C atom ratio were based on the integral of the charging current, corrected for the background capacitive contribution of the Pt plate electrode in control experiments. Raman spectra of powder/drop-casted samples were obtained with a LabRAM Infinity instrument (Horiba Jobin-Yvon Ltd) with a 633 nm He-Ne laser (1.96 eV) and 532 nm Nd-YAG laser (2.33 eV). All Raman spectra were recorded using a grating of 1,800 grooves per mm. The maximum powers of the 633 and 532 nm lasers at the sample were 8 and 24 mW, respectively. The laser power was varied to ensure no damage to samples; typically, 100% intensity was used for the 633 nm laser, 25% intensity for the 532 nm laser. Samples were measured either in raw powder form or as drop-casted dispersions on glass microscope slides. At least five consistent spectra were measured for each sample at different locations to reduce the effect of sample heterogeneity. TEM was carried out using a JEOL2010 TEM operating at 200 kV. Samples were prepared on 300 copper mesh holey carbon grids (Agar Scientific) by drop casting on to the grid supported by a filter paper, and left to dry in a nitrogen-filled glove box for several days. Samples were vacuum dried at room temperature to remove PC for 24 h, washed on filter paper with 2–3 drops of PC to remove electrolytic salts, then further washed with IPA. Atomic force microscopy was carried out using a Bruker Multimode 8 AFM with Nanoscope V controller in tapping mode using samples prepared as above. UV–vis absorption spectroscopy was carried out using a Lambda 950 spectrophotometer (Perkin-Elmer). Concentrations and hence yields were estimated using a typical SWCNT extinction coefficient [22] (3,264 ml mg −1 m −1 at 660 nm). As-received SWCNT dispersions (for control experiments) were produced using a 750-W ultrasonic processor (Sonics and Materials Inc, CT, USA). Subsequent ultracentrifugation was carried out using a Beckmann Coulter Optima L-90 K with swinging bucket rotor (SW-41Ti). How to cite this article: Hodge, S. A. et al . Giant cationic polyelectrolytes generated via electrochemical oxidation of single-walled carbon nanotubes. Nat. Commun. 4:1989 doi: 10.1038/ncomms2989 (2013).